Functional annotation of colon cancer risk SNPs Colorectal cancer (CRC) is a leading cause of cancer-related deaths in the United States. Genome-wide association studies (GWAS) have identified single nucleotide polymorphisms (SNPs) associated with increased risk for CRC. A molecular understanding of the functional consequences of this genetic variation has been complicated because each GWAS SNP is a surrogate for hundreds of other SNPs, most of which are located in non-coding regions. Here we use genomic and epigenomic information to test the hypothesis that the GWAS SNPs and/or correlated SNPs are in elements that regulate gene expression, and identify 23 promoters and 28 enhancers. Using gene expression data from normal and tumour cells, we identify 66 putative target genes of the risk-associated enhancers (10 of which were also identified by promoter SNPs). Employing CRISPR nucleases, we delete one risk-associated enhancer and identify genes showing altered expression. We suggest that similar studies be performed to characterize all CRC risk-associated enhancers. Colorectal cancer (CRC) ranks among the leading causes of cancer-related deaths in the United States. The incidence of death from CRC is in the top 3 of all cancers in the United States for both men and women ( http://apps.nccd.cdc.gov/uscs/toptencancers.aspx ). It is estimated that 142,820 men and women will be diagnosed with, and 50,830 men and women will die of, cancer of the colon and rectum in 2013 ( http://seer.cancer.gov/-statfacts/html/colorect.html ). A better understanding of the regulatory factors and signalling pathways that are deregulated in CRC could provide new insights into appropriate chemotherapeutic targets. Decades of studies have revealed that certain genes and pathways, such as WNT, RAS, PI3K, TGF-B, p53 and mismatch repair proteins, are important in the initiation and progression of CRC [1] . In an attempt to obtain a more comprehensive view of CRC, two new approaches have been used: exome sequencing of tumours and genome-wide population analyses of human variation. The Cancer Genome Atlas (TCGA) has taken the first of these new approaches in the hopes of moving closer to a full molecular characterization of the genetic contributions to CRC, analyzing somatic alterations in 224 tumours [2] . These studies again implicated the WNT, RAS and PI3K signalling pathways. The second new approach identifies single nucleotide polymorphisms (SNPs) associated with specific diseases using genome-wide association studies (GWAS). GWAS has led to the identification of thousands of SNPs associated with a large number of phenotypes [3] , [4] . Such studies identify what are known as tag SNPs that are associated with a particular disease. Specifically for CRC, 25–30 tag SNPs have been identified [5] , [6] , [7] , [8] , [9] , [10] , [11] , [12] . Although identification of tag SNPs is an important first step in understanding the relationship between human variation and risk for CRC, a major challenge in the post-GWAS era is to understand the functional significance of the identified SNPs [13] . It is critical to advance the field by progressing from a statistical association between genetic variation and disease to a molecular understanding of the functional consequences of the genetic variation. Progress towards this goal has been mostly successful when the genetic variation falls within a coding region. Unfortunately, most SNPs identified as associated with human disease in large GWAS studies are located within large introns or distal to coding regions, in what in the past has been considered to be the unexplored territory of the genome. However, recent studies from the ENCODE Consortium have shown that introns and regions distal to genes contain regulatory elements. In particular, the ENCODE Consortium has made major progress in defining hundreds of thousands of cell-type-specific distal enhancer regions [14] , [15] , [16] . Comparison of GWAS SNPs to these enhancer regions has revealed several important findings. For example, work from ENCODE and others [13] , [15] , [17] , [18] have shown that many GWAS SNPs fall within enhancers, DNase hypersensitive sites and transcription factor binding sites. It is also clear that the SNP whose functional role is most strongly supported by ENCODE data is often a SNP in linkage disequilibrium (LD) with the GWAS tag SNP, not the actual SNP reported in the association study [19] . These recent reports clearly show that regulatory elements can help to identify important SNPs [13] , [19] , [20] . However, the studies were performed using all available ENCODE data and did not focus the functional analysis of cancer-associated SNPs on the regulatory information obtained using the relevant cell types. Using epigenetic marks obtained from normal colon and colon cancer cells, we identify SNPs in high LD with GWAS SNPs that are located in regulatory elements specifically active in normal and/or tumour colon cells. Characterization of transcripts nearby CRC risk-associated promoters and enhancers using RNA expression data allows the prediction of putative genes and non-coding RNAs associated with an increased risk of colon cancer. Using genomic nucleases, we delete one risk-associated enhancer and compare the deregulated genes with those predicted to be targets of that enhancer. Our studies suggest that transcriptome characterization after precise deletion of a risk-associated enhancer could be a useful approach for post-GWAS analyses. 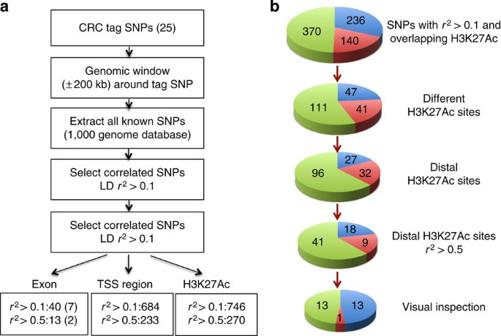Figure 1: Identification of potential functional SNPs for CRC. (a) Shown is the number of SNPs identified by FunciSNP in each of three categories for 25 colon cancer risk loci (seeTable 1for information on each CRC risk SNP). For exons, only non-synonymous SNPs are reported; parentheses indicated the number of SNPs that are predicted to be damaging; seeTable 2for a list of the expressed genes associated with the correlated SNPs. For TSS regions, the region from −2 kb to +2 kb relative to the start site of all transcripts annotated in GENCODE V15, including coding genes and non-coding RNAs was used; seeTable 2for a list of expressed transcripts associated with the correlated SNPs. (b) For H3K27Ac analyses, ChIP-seq data from normal sigmoid colon and HCT116 tumour cells were used; seeTable 3for further analysis of distal regions harbouring SNPs in normal and tumour colon cells. The SNPs having anr2>0.1 that overlapped with H3K27Ac sites were identified separately for HCT116 and sigmoid colon data sets. Because more than one SNPs could identify the same H3K27Ac-marked region, the SNPs were then collapsed into distinct H3K27Ac peaks. The sites that were within ±2 kb of a promoter region were removed to limit the analysis to distal elements. To obtain a more stringent set of enhancers, those regions having only SNPs withr2<0.5 were removed. This remaining set of 68 distal H3K27Ac sites were contained within 19 of the 25 risk loci. Visual inspection to identify only the robust enhancers having linked SNPs not at the margins reduced the set to 27 enhancers located in 9 of the 25 risk loci; an additional enhancer was identified in SW480 cells (seeTable 3for the genomic locations of all 28 enhancers). Colour key: green=SNPs or H3K27Ac sites unique to normal colon, red=unique to colon tumour cells, blue=present in both normal and tumour colon. CRC risk-associated SNPs linked to a specific gene For our studies, we chose 25 tag SNPs, 4 of which have been associated with an increased risk for CRC in Asia-derived case-control cohorts and the rest in Europe-derived case-control cohorts; the genomic coordinates of each SNP can be found in Table 1 and Supplementary Data 1 . Of these 25 tag SNPs, only one is found within an exon, occurring in the third exon of the MYNN gene and resulting in a synonymous change that does not lead to a coding difference. However, there are hundreds of SNPs in high LD with each tag SNP and it is possible that some of the high LD SNPs may reside in coding exons. To address this possibility we used a bioinformatics programme called FunciSNP to identify SNPs correlated with CRC tag SNPs that also intersect the set of coding exons in the human genome [21] . FunciSNP is an R/Bioconductor package that allows a comparison of population-based correlated SNPs from the 1,000 Genomes Project ( http://www.1000genomes.org/ ) with any set of chromatin biofeatures. In this initial analysis, we chose coding exons from the Gencode 15 data set ( http://www.gencodegenes.org/releases/ ) as the biofeature. Because LD varies with the population, to identify population-based correlated SNPs we specified the Asian population for analysis of the four tag SNPs identified using Asian-derived case-control cohorts and we specified the European population for analysis of the rest of the tag SNPs. Using FunciSNP, we identified 240 unique SNPs that are correlated with the 25 tag SNPs at an r 2 >0.1 and are within a coding exon ( Supplementary Fig. 1 ). We then used snpeff ( http://snpeff.sourceforge.net/ (ref. 22 )) to determine that 40 of these correlated SNPs create non-synonymous changes; however, limiting the SNPs to those with an LD of r 2 >0.5 with the tag SNP reduced the number to only 13. Using polyphen-2 ( http://genetics.bwh.harvard.edu/pph2/ (ref. 23 )) and provean ( http://provean.jcvi.org/index.php (ref. 24 )), only two potentially damaging SNPs at r 2 >0.5 were found, both in POU5F1B ( Fig. 1 ). At the less restrictive r 2 >0.1, four other genes were also found to harbour a damaging SNP ( RHPN2 , UTP23 , LAMA5 and FAM186A ). To determine if these genes are expressed in colon cells, we performed two replicates of RNA-seq for HCT116 cells and also used RNA-seq data from the Roadmap Epigenome Mapping Consortium for normal sigmoid colon to examine expression. After analysis of both sets of RNA-seq data, we categorized transcripts that are not expressed as having <0.5 FPKM (expected fragments per kilobase of transcripts per million fragments sequenced) ( Supplementary Fig. 2 ). 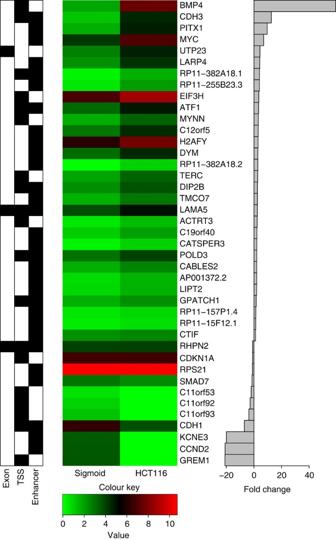Figure 2: Expression of risk-associated genes in colon cells. The left panel indicates if a transcript was identified by a SNP located in an exon or a TSS or is nearby a risk-associated enhancer; the middle panel shows the expression values of each of the 41 transcripts in sigmoid colon or HCT116 tumour cells; the right panel shows the fold change of each transcript in the tumour cells (positive indicates higher expression in the tumour). Analysis of the RNA-seq data revealed that POU5F1B and FAM186A are not expressed in either the normal sigmoid colon or HCT116 cells (however, these genes are expressed in a cohort of TCGA colon tumours; see Table 2 ). Table 1 Summary of regions linked to CRC tag SNPs. Full size table Figure 1: Identification of potential functional SNPs for CRC. ( a ) Shown is the number of SNPs identified by FunciSNP in each of three categories for 25 colon cancer risk loci (see Table 1 for information on each CRC risk SNP). For exons, only non-synonymous SNPs are reported; parentheses indicated the number of SNPs that are predicted to be damaging; see Table 2 for a list of the expressed genes associated with the correlated SNPs. For TSS regions, the region from −2 kb to +2 kb relative to the start site of all transcripts annotated in GENCODE V15, including coding genes and non-coding RNAs was used; see Table 2 for a list of expressed transcripts associated with the correlated SNPs. 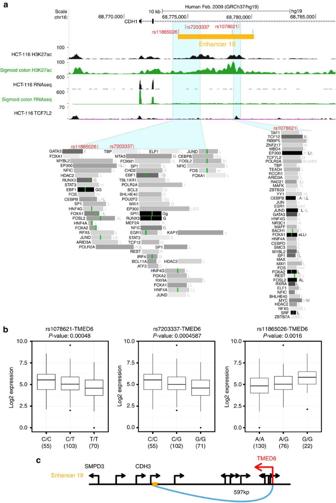Figure 3: Linking a transcript to an enhancers using TCGA data. (a) Shown is the location of enhancer 19 and the position of the three SNPs (in red) identified in the eQTL studies and two other SNPs (in blue) identified by the FunciSNP analysis but not present on the SNParray, in relation to the H3K27Ac, RNA-seq and TCF7L2 ChIP-seq data for that region. Also shown are the ENCODE ChIP-seq transcription factor tracks from the University of California, Santa Cruz genome browser. (b) The expression of theTMED6RNA is shown for samples having homozygous or heterozygous alleles for three SNPs in enhancer 19. The upper and lower quartiles of the box plots are the 75th and 25th percentiles, respectively. The whisker top and bottom are 90th and 10th percentiles, respectively. The horizontal line through the box is median value. TheP-value corresponds to the regression coefficient based on the residue expression level and the germline genotype. Sample size is listed under each genotype. (c) A schematic of the gene structure in the genomic region around enhancer 19 (yellow box) is shown; the arrows indicate the direction of transcription of each gene. The three genes in the enhancer 19 region that showed differential expression in normal versus tumour colon samples (Table 5) are indicated; of these, onlyTMED6was identified in the eQTL analysis. ( b ) For H3K27Ac analyses, ChIP-seq data from normal sigmoid colon and HCT116 tumour cells were used; see Table 3 for further analysis of distal regions harbouring SNPs in normal and tumour colon cells. The SNPs having an r 2 >0.1 that overlapped with H3K27Ac sites were identified separately for HCT116 and sigmoid colon data sets. Because more than one SNPs could identify the same H3K27Ac-marked region, the SNPs were then collapsed into distinct H3K27Ac peaks. The sites that were within ±2 kb of a promoter region were removed to limit the analysis to distal elements. To obtain a more stringent set of enhancers, those regions having only SNPs with r 2 <0.5 were removed. This remaining set of 68 distal H3K27Ac sites were contained within 19 of the 25 risk loci. Visual inspection to identify only the robust enhancers having linked SNPs not at the margins reduced the set to 27 enhancers located in 9 of the 25 risk loci; an additional enhancer was identified in SW480 cells (see Table 3 for the genomic locations of all 28 enhancers). Colour key: green=SNPs or H3K27Ac sites unique to normal colon, red=unique to colon tumour cells, blue=present in both normal and tumour colon. Full size image Table 2 Expressed transcripts directly linked to CRC tag SNPs. Full size table Another way to link a SNP to particular gene is if the SNP falls within a promoter region. We again used FunciSNP, but this time the biofeature analyzed corresponded to the region from −2,000 to +2,000 nucleotides of the transcription start site (TSS) of each transcribed gene (we analyzed coding and non-coding transcripts from GENCODE V15). We chose to include 2 kb upstream and downstream of the start site as the promoter-proximal regions because several studies [25] , [26] , as well as visual inspection of the ENCODE TF Chromatin Immunoprecipitation sequencing (ChIP-seq) tracks, have shown that transcription factors can bind on either side of a TSS. Using an r 2 >0.1, we found 684 correlated promoter SNPs which were reduced to 233 SNPs at r 2 >0.5 ( Fig. 1 and Supplementary Fig. 3 ). Many of these SNPs fall within the same promoter regions. When collapsed into distinct promoters, we identified the TSS regions of 17 protein-coding genes and 2 non-coding RNAs which are expressed in HCT116 or sigmoid colon cells; promoter SNPs identified 4 additional expressed genes when a larger number of TCGA colon tumour samples were analyzed ( Table 2 ). CRC risk-associated SNPs in distal regulatory regions Most of the SNPs in LD with the CRC GWAS tag SNPs cannot be easily linked to a specific gene because they do not fall within a coding region or a promoter-proximal region. However, it is possible that a relevant SNP associated with increased risk lies within a distal regulatory element of a gene whose function is important in cell growth or tumorigenicity. To address this possibility, we used the histone modification H3K27Ac to identify active regulatory regions throughout the genome of colon cancer cells or normal sigmoid colon cells. We used HCT116 H3K27Ac ChIP-seq data [16] produced in our lab for the tumour cells and we obtained H3K27Ac ChIP-seq data for normal colon cells from the NIH Roadmap Epigenome Mapping Consortium. The ChIP-seq data for both the normal and tumour cells included two replicates. To demonstrate the high quality of the data sets, we called peaks on each replicate of H3K27Ac from HCT116 and each replicate of H3K27Ac from sigmoid colon using Sole-search [27] , [28] and compared the peak sets from the two replicates using the ENCODE 40% overlap rule (after truncating both lists to the same number, 80% of the top 40% of one replicate must be found in the other replicate and vice versa ). After determining that the HCT116 and sigmoid colon data sets were of high quality ( Supplementary Fig. 4 ), we merged the two replicates from HCT116 and separately merged the two replicates from sigmoid colon and called peaks on the two merged data sets; see Supplementary Data 2 for a list of all ChIP-seq peaks. Using the merged peak lists from each of the samples as biofeatures in FunciSNP, we determined that 746 of the 4,894 SNPs that were in LD with a tag SNP at r 2 >0.1 were located in H3K27Ac regions identified in either the HCT116 or sigmoid colon peak sets; of these 270 SNPs had an r 2 >0.5 with a tag SNP ( Fig. 1 and Supplementary Fig. 5 ). A comparison of the H3K27Ac peaks from normal and tumour cells indicated that the patterns are very similar; in fact, ~24,000 H3K27Ac peaks are in common in the normal and tumour cells. However, there are clearly some peaks unique to normal and some peaks unique to the tumour cells. Therefore, we separately analyzed the normal and tumour H3K27Ac ChIP-seq peaks as different sets of biofeatures using FunciSNP ( Fig. 1b ). Of the 746 SNPs, 236 were located in a H3K27Ac site common to both normal and tumour cells, whereas 140 were unique to tumour and 370 were unique to normal cells. Visual inspection of the SNPs and peaks using the University of California, Santa Cruz (UCSC) genome browser showed that many of the identified enhancers harboured multiple correlated SNPs. Reduction of the number of SNPs to the number of different H3K27Ac sites resulted in 47 common, 41 tumour-specific and 111 normal-specific regions. Visual inspection also showed that some of the H3K27 genomic regions corresponded to promoter regions ( Supplementary Fig. 4 ). Because promoter regions having correlated SNPs were already identified using TSS regions (see above), we eliminated the promoter-proximal H3K27Ac sites, resulting in 27 common, 32 tumour-specific and 96 normal-specific distal H3K27Ac regions. As the next winnowing step, we selected only those enhancers having at least one SNP with an r 2 >0.5, leaving 18 common, 9 tumour-specific and 41 normal-specific distal H3K27Ac regions. We noted that some of the identified regions corresponded to low-ranked H3K27Ac peaks. For our subsequent analyses, we wanted to limit our studies to robust enhancers that harbour correlated SNPs. Therefore, we visually inspected each of the genomic regions identified as having distal H3K27Ac peaks harbouring a correlated SNP. To prioritize the distal regions for further analysis, we eliminated those for which the correlated SNPs was on the edge of the region covered by the H3K27Ac signal or corresponded to a very low-ranked peak. After inspection, we were left with a set of 27 distal H3K2Ac regions in which a correlated SNP ( r 2 >0.5) was well within the boundaries of a robust peak ( Fig. 1b ). To confirm our results, we repeated the analysis using H3K27Ac data from a different colon cancer cell line, SW480, identifying only one additional enhancer harbouring risk SNPs for CRC. The genomic coordinates of each of these 28 enhancers, which are clustered in nine genomic regions, are listed in Table 3 (see also Supplementary Table 1 ). Combining all data, enhancers in five of the nine regions were identified in all three cell types and eight of the nine regions were identified in at least two of the cell types. Table 3 Distal regulatory regions correlated with CRC tag SNPs. Full size table Effects of SNPs on binding motifs in the distal elements To determine possible effects of the correlated SNPs on transcription factor binding, we first analyzed all SNPs having an r 2 >0.1 with the 25 CRC tag SNPs. Using position weight matrices from Factorbook [29] , all correlated SNPs that fell within a critical position in a transcription factor binding motif were identified ( Supplementary Data 3 ). We identified ~800 SNPs that were predicted to impact binding of transcription factor to a known motif. However, most of these SNPs are not in regulatory regions important for CRC. Therefore, we next limited our analysis to the set of correlated SNPs that fall within the 28 robust enhancers ( Supplementary Table 2 ). We found 80 SNPs that cause motif changes in a total of 124 motifs, representing binding sites for 40 different transcription factors. 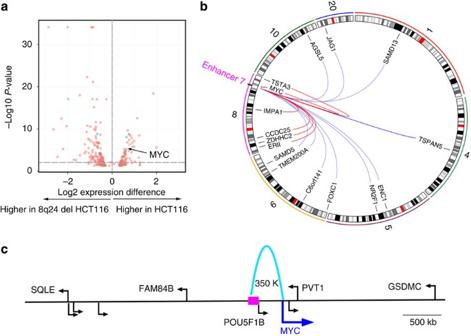Figure 4: Identification of genes affected by deletion of enhancer 7. (a) Shown are the expression differences (xaxis) and the significance of the change (y axis) of the genes in the control HCT116 versus HCT116 cells having complete deletion of enhancer 7. The Illumina Custom Differential Expression Algorithm was used to determineP-values to identify the significantly altered genes; three replicates each for the control and deleted cells were used. Genes on chromosome 8 (the location of enhancer 7) are shown in blue. The spot representing theMYCgene is indicated by the arrow. (b) Shown are all genes on chromosome 8 that change in expression and the 10 genes showing the largest changes in expression upon deletion of enhancer 7. The location of the enhancer is indicated and the chromosome number is shown on the outside of the circle. (c) The genes identified as potential targets using TCGA expression data are indicated; of these,MYCis the only showing a change in gene expression upon deletion of the enhancer. Using RNA-seq data, we found that 36 of these factors are expressed in HCT116 and/or sigmoid colon cells ( Table 4 ), suggesting that perhaps the binding of these factors at the risk-associated enhancers is influenced by the correlated SNPs. Of the 36 factors, most were expressed at either approximately the same levels in normal and tumour colon or at higher levels in HCT116 cells than in normal colon. However, several factors showed large decreases in gene expression in HCT116 as compared with sigmoid colon cells, including FOS and JUN which were ~10-fold higher in normal colon and HNF4A and ETS1 which were 30–40-fold higher in normal colon; Supplementary Table 3 . Table 4 Effects of SNPs on motifs in the distal regulatory regions. Full size table Expression analysis of candidate risk-associated genes Although the genes identified by the exon or TSS SNPs are clearly good candidate genes for analysis of their possible role in the development of colon cancer, it is difficult to definitively link a target gene with a distal enhancer region because enhancers can function in either direction and do not necessarily regulate the nearest gene. In fact, the ENCODE Consortium recently reported that, on an average, a distal element can physically associate with approximately three different promoter regions [30] . Also, only 27% of the distal elements showed an interaction with the nearest TSS, although this increased to 47% when only expressed genes were used in the analysis [30] . Taken together, these analyses suggest that examining the three nearest genes may produce a reasonable list of genes potentially regulated by the CRC risk-associated enhancers. Therefore, we used the GENCODE V15 data set and identified the three nearest promoters of coding genes and three nearest promoters of non-coding transcripts around each of the 28 enhancers ( Supplementary Table 1 ). We next limited the nearby coding and non-coding transcripts to those expressed in either sigmoid colon RNA or HCT116 cells ( Table 3 ); we note that taking into account expression did not greatly change the list of coding transcripts but eliminated most of the non-coding transcripts, which tend to be expressed in a very cell-type-specific manner. Interestingly, several of the genes nearby the risk-associated enhancers were also identified in the TSS analyses, suggesting that a putative causal gene associated with CRC might be differentially regulated by risk-associated SNPs found in the promoter and in a nearby enhancer ( Fig. 2 ). We note that in these cases, the promoters and enhancers were identified by different risk-associated SNPs in high LD with a tag SNP, with the promoters being identified by SNPs within ±2 kb of the TSS and enhancers being identified by distal SNPs. We further analyzed the expression levels of all genes directly linked to the risk SNPs (by exons or TSS) and the expressed genes nearby the risk-associated enhancers in normal colon and HCT116 tumour cells. Shown in Fig. 2 are the expression levels of each of the 41 transcripts and the fold change in expression in HCT116 versus normal cells; several of these genes display robust changes in expression in the tumour cells. Figure 2: Expression of risk-associated genes in colon cells. The left panel indicates if a transcript was identified by a SNP located in an exon or a TSS or is nearby a risk-associated enhancer; the middle panel shows the expression values of each of the 41 transcripts in sigmoid colon or HCT116 tumour cells; the right panel shows the fold change of each transcript in the tumour cells (positive indicates higher expression in the tumour). Full size image As a second approach to identify transcripts potentially regulated by the identified enhancers, we developed a new statistical approach that employs RNA-seq data from TCGA. We selected the 10 nearest genes 5′ of and the 10 nearest genes 3′ of each of the 28 enhancers. Because of the difference in gene density in different regions of the genome, the 20-gene span ranged from 786 kb to 7.5 MB, depending on the specific enhancer. Because several of the 28 enhancers are clustered near each other, this resulted in a total of 182 unique genes. We downloaded the RNA-seq data for 233 colorectal tumour samples and 21 colorectal normal samples from the TCGA data download website ( https://tcga-data.nci.nih.gov/tcga/dataAccessMatrix.htm ) and determined if any of the 182 genes show a significant increase or decrease (greater than twofold change and P -value <0.01) in colon tumours versus normal colon (see Methods and Supplementary Fig. 6 for an analysis of potential TCGA batch effects). 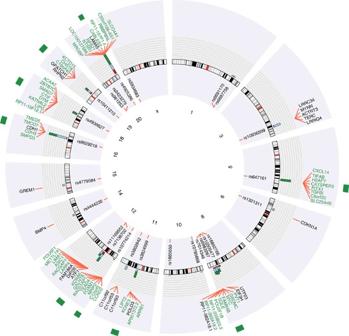Figure 5: Summary of identified candidate genes correlated with increased risk for CRC. Shown are the 80 candidate genes identified in this study. For the gene names, green means that it was only identified as a potential enhancer target, the other genes were identified as direct targets either by an exon SNP or a TSS SNP; the putative enhancer target genes were selected as described in the text. For each tag SNP, the relative number of SNPs that identified an exon (red portion), a TSS (blue portion), or an enhancer (green portion) is shown by the bar graph. The nine genomic regions that harbour CRC risk enhancers are shown by the green rectangles outside the circle. We then eliminated those genes whose expression change did not correspond to the nature of the enhancer (for example, a tumour-specific enhancer should not regulate a gene that is higher in normal cells), leaving a total of 39 possible genes whose expression might be differentially regulated in colon cancer by the risk enhancers ( Table 5 ). We note that five of the genes shown to be differentially expressed in the TCGA data ( MYC , PITX1 , POU5F1B , C5orf20 and CDH3 ) are also in the set of the nearest three genes to an enhancer having CRC risk-associated SNPs. We found that 0–6 differentially expressed genes were linked to an enhancer using the TCGA data, with an average of 4 transcripts per enhancer that showed correct differential expression in colon tumours. Heatmaps of the expression of the 39 putative enhancer-regulated genes, as well as the expression of the genes identified by exon and promoter SNPs, in the TCGA samples are shown in Supplementary Fig. 7 . To determine if we could validate any of the putative enhancer targets, we used expression quantitative trait loci (eQTL) analyses based on data from TCGA. We began by identifying the SNPs within each of the 28 enhancers that are on the Illumina WG SNP6 array used by TCGA. Unfortunately, these arrays include only 8% of the SNPs of interest (that is, the exon, promoter and enhancer SNPs that are correlated with the CRC tag SNPs), greatly limiting our ability to effectively utilize the eQTL methodology. However, we did identify two examples of allelic expression differences in the set of putative enhancer targets that correlated with SNPs in an enhancer region. Both of these SNPs fell within enhancer 19 and showed correlation with allelic expression differences of the TMED6 gene (the two SNPs significantly associated with TMED6 expression had an adjusted P -value False Discovery Rate (FDR)<0.1 for rs7203339 and rs1078621); enhancer 19 falls within the intron of the CDH1 gene, which is 600 kb from the TSS of the TMED6 gene ( Fig. 3 ). A summary of the eQTL analysis of enhancer and promoter risk-associated SNPs can be found in Supplementary Data 4 and Supplementary Fig. 8 . Table 5 Linking transcripts to enhancers using TCGA data. Full size table Figure 3: Linking a transcript to an enhancers using TCGA data. ( a ) Shown is the location of enhancer 19 and the position of the three SNPs (in red) identified in the eQTL studies and two other SNPs (in blue) identified by the FunciSNP analysis but not present on the SNParray, in relation to the H3K27Ac, RNA-seq and TCF7L2 ChIP-seq data for that region. Also shown are the ENCODE ChIP-seq transcription factor tracks from the University of California, Santa Cruz genome browser. ( b ) The expression of the TMED6 RNA is shown for samples having homozygous or heterozygous alleles for three SNPs in enhancer 19. The upper and lower quartiles of the box plots are the 75th and 25th percentiles, respectively. The whisker top and bottom are 90th and 10th percentiles, respectively. The horizontal line through the box is median value. The P -value corresponds to the regression coefficient based on the residue expression level and the germline genotype. Sample size is listed under each genotype. ( c ) A schematic of the gene structure in the genomic region around enhancer 19 (yellow box) is shown; the arrows indicate the direction of transcription of each gene. The three genes in the enhancer 19 region that showed differential expression in normal versus tumour colon samples ( Table 5 ) are indicated; of these, only TMED6 was identified in the eQTL analysis. Full size image The effect of enhancer deletion on the transcriptome The expression analyses described above provide a list of genes that potentially are regulated by the CRC risk-associated enhancers. However, it is possible that the enhancers regulate only a subset of those genes and/or the target genes are at a greater distance than was analyzed. One approach to identify targets of the CRC risk-associated enhancers would be to delete an enhancer from the genome and determine changes in gene expression. As an initial test of this method, we selected enhancer 7, located at 8q24. The region encompassing this enhancer has previously been implicated in regulating expression of MYC [31] , which is located 335 kb from enhancer 7. We introduced guide RNAs that flanked enhancer 7, along with Cas9, into HCT116 cells, and identified cells that showed deletion of the enhancer. We then performed expression analysis using gene expression arrays, identifying 105 genes whose expression was downregulated in the cells having a deleted enhancer ( Supplementary Data 5 ); the closest one was MYC , which was expressed 1.5 times higher in control versus deleted cells ( Fig. 4 ). Figure 4: Identification of genes affected by deletion of enhancer 7. ( a ) Shown are the expression differences ( x axis) and the significance of the change (y axis) of the genes in the control HCT116 versus HCT116 cells having complete deletion of enhancer 7. The Illumina Custom Differential Expression Algorithm was used to determine P -values to identify the significantly altered genes; three replicates each for the control and deleted cells were used. Genes on chromosome 8 (the location of enhancer 7) are shown in blue. The spot representing the MYC gene is indicated by the arrow. ( b ) Shown are all genes on chromosome 8 that change in expression and the 10 genes showing the largest changes in expression upon deletion of enhancer 7. The location of the enhancer is indicated and the chromosome number is shown on the outside of the circle. ( c ) The genes identified as potential targets using TCGA expression data are indicated; of these, MYC is the only showing a change in gene expression upon deletion of the enhancer. Full size image We have used the programme FunciSNP [21] , in combination with genomic, epigenomic and transcriptomic data, to analyze 25 tag SNPs (and all SNPs in high LD with those tag SNPs) that have been associated with an increased risk for CRC [5] , [6] , [7] , [8] , [9] , [10] , [11] , [12] . Taken together, we have identified a total of 80 genes that may be regulated by risk-associated SNPs. Of these, 24 are directly linked to a gene via a SNP within an exon or proximal promoter region and 56 additional genes are putative target genes of risk-associated enhancers; see Fig. 5 for a schematic summary of the location of the tag and LD SNPs and associated genes, and Supplementary Table 4 for a complete list of genes and how they were identified. Figure 5: Summary of identified candidate genes correlated with increased risk for CRC. Shown are the 80 candidate genes identified in this study. For the gene names, green means that it was only identified as a potential enhancer target, the other genes were identified as direct targets either by an exon SNP or a TSS SNP; the putative enhancer target genes were selected as described in the text. For each tag SNP, the relative number of SNPs that identified an exon (red portion), a TSS (blue portion), or an enhancer (green portion) is shown by the bar graph. The nine genomic regions that harbour CRC risk enhancers are shown by the green rectangles outside the circle. Full size image Of the 25 tag SNPs, only one is found within a coding exon, occurring in the third exon of the MYNN gene and resulting in a synonymous change that does not lead to a coding difference. However, by analysis of SNPs in high LD with the 25 tag SNPs, we identified five genes that harbour damaging SNPs and which are expressed in colon cells (HCT116, normal sigmoid colon or TCGA tumours); these are POU5F1B , RHNP2 , UTP23 , LAMA5 and FAM186A ). Interestingly, the retrogene POU5F1B which encodes a homologue of the stem cell regulator OCT4 has recently been associated with prostate cancer susceptibility [32] . We also identified 23 genes (21 coding and 2 non-coding) that harbour highly correlated SNPs in their promoter regions and are expressed in colon cells. Several of the genes that we have linked to increased risk for CRC by virtue of promoter SNPs show large changes in gene expression in tumour versus normal colon tissue. For example, TERC , the non-coding RNA that is a component of the telomerase complex, was identified by a promoter SNP and has higher expression in a subset of colon tumours ( Supplementary Fig. 7A ). Similarly, CDH3 (P-cadherin) was identified by a promoter SNP and shows increased expression in many of the colon tumours. Both TERC and CDH3 have previously been linked to cancer [33] , [34] . Promoter SNPs also identified three uncharacterized protein-coding genes ( c11orf93 , c11orf92 and c11orf53 ) clustered together on chromosome 11. Inspection of H3K4me3 and H3K27Ac ChIP-seq signals suggested that these genes are in open chromatin in normal sigmoid colon, but not in HCT116. Accordingly, the TCGA gene expression data showed that all three genes are downregulated in a subset of human CRC tumours ( Supplementary Fig. 7A ). Additional genes identified by promoter SNPs that have been linked to cancer include ATF1 , BMP4 , CDH1 , CDKN1A , EIF3H , GREM1 , LAMA5 and RHPN2 (refs 34 , 35 , 36 , 37 , 38 , 39 , 40 , 41 , 42 , 43 , 44 , 45 ). For example, BMP4 is upregulated in the HCT116 cells and has been suggested to confer an invasive phenotype during progression of colon cancer [41] . Interestingly, we also identified GREM1 , an antagonist of BMP proteins, and showed that expression of GREM1 is decreased in HCT116. The downregulation of the antagonist GREM1 and the upregulation of the cancer-promoting BMP4 may cooperate to drive colon cancer progression. LAMA5 is a subunit of laminin-10, laminin-11 and laminin-15. Laminins, a family of extracellular matrix glycoproteins, are the major non-collagenous constituent of basement membranes and have been implicated in a wide variety of biological processes including cell adhesion, migration, signalling and metastasis [46] . We identified 28 enhancers, clustered in 9 genomic regions, that harbour correlated SNPs. It is important to note that in our studies we have used the appropriate cell types and the appropriate epigenetic mark to identify CRC-associated enhancers. Previous analyses have attempted to link SNPs to enhancers by using transcript abundance, epigenetic marks or transcription factor binding from non-colon cell types [47] . In contrast, we have used normal and tumour cells from the colon. Of equal importance is the actual epigenetic mark that is used to identify enhancers. A previous study used H3K4me1 to identify genomic regions that were differently marked between normal and tumour colon cells [18] . However, although H3K4me1 is associated with enhancer regions, this mark does not specifically identify active enhancers. Some regions marked by H3K4me1 are classified as ‘weak’ or ‘poised’ enhancers and it is thought that these regions may become active in different cells or developmental states [48] . In contrast, H3K27Ac is strongly associated with active enhancers [49] , [50] and we feel that this mark is the most appropriate one for identification of CRC-associated risk enhancers. Although it is not possible to conclusively know a priori what gene is regulated by each of the identified enhancers, we have derived a list of putative CRC risk-associated enhancer target genes by examining gene expression data from HCT116 cells and from a large number of colon tumours. Several of the genes that are possible enhancer targets are transcription factors that have previously been linked to cancer, including H2AFY, MYC, SMAD7, PITX1, TEAD4 and ZBTB7C. MYC, of course, has been linked to colon cancer by many studies due to the fact that it is a downstream mediator of WNT signalling, which is strongly correlated with colon cancer [2] . In addition, PITX1, TEAD4 and ZBTB7C are all transcription factors that have been previously linked to the control of cell proliferation, specification of cell fate or regulation of telomerase activity [51] , [52] , [53] , [54] . Also, PVT1 is a MYC-regulated non-coding RNA that may play a role in neoplasia [55] , [56] . In conclusion, we have used epigenomic and transcriptome information from normal and tumour colon cells to identify a set of genes that may be involved in an increased risk for the development of colon cancer. We realize that we cast a rather large net by analyzing 10 genes 5′ and 10 genes 3′ of each enhancer. We note that five of the genes shown to be differentially expressed in the TCGA data ( MYC , PITX1 , POU5F1B , C5orf20 and CDH3 ) are also in the set of nearest three genes to an enhancer having CRC risk-associated SNPs. However, enhancers can also work at large distances. In fact, the eQTL analysis identified TMED6 as a potential target of enhancer 19 (over 600 kb away) and deletion of enhancer 7 identified MYC as a potential target (335 kb away). Future analyses of the entire set of CRC risk-associated enhancers are required to confirm the additional putative long range regulatory loops suggested by our studies. Such studies will provide a high confidence list of genes which, when combined with the genes identified by the TSS risk-associated SNPs, should be prioritized for analysis in tumorigenicity assays. RNA-seq RNA-seq data was downloaded from the Reference Epigenome Mapping Center for analysis of gene expression in sigmoid colon cells (GSM1010974 and GSM1010942). For HCT116 colon cancer cells, RNA was prepared using Trizol (Life Technologies, Carlsbad, CA, USA), paired-end libraries were prepared using the Illumina TruSeqV2 Sample Prep Kit (Catalogue# 15596-026), starting with 1 μg total RNA. Libraries were barcoded, pooled and sequenced using an Ilumina Hiseq. For analysis of RNA-seq data, we used Cufflinks [57] , a programme of ‘alignment to annotation’ having discontinuous mapping to the reference genome. Messenger RNA (mRNA) abundance was measured by calculating FPKM, to allow inter-sample comparisons. We specified the –G option with the GENCODE V15 comprehensive annotation so that the programme will only do alignments that are structurally compatible with the reference transcript provided. Two biological replicates were performed and the mean FPKM of two biological replicates represents the expression of each gene (GSM1266733 and GSM1266734). We categorized genes into non-expressed, low expressed and expressed based on the distribution of the Gene FPKM ( Supplementary Fig. 2 ) generated by the R package ‘ggplot2’. RNA-seq data for 233 colorectal tumour samples and 21 colorectal normal samples were downloaded from the TCGA data download website ( https://tcga-data.nci.nih.gov/tcga/dataAccessMatrix.htm ); Supplementary Data 6 . The data were all generated on the Illumina HiSeq platform, and mapped with the RSEM algorithm and normalized so that the third quartile for each sample equals 1,000. Entrez gene IDs were used for mapping to genomic locations using GenomicRanges ( http://www.bioconductor.org/packages//2.12/bioc/html/GenomicRanges.html ). To identify transcripts differentially expressed in the tumour samples, we selected the 10 nearest genes 5′ of and the 10 nearest genes 3′ of each of the 28 enhancers. After removing the non-expressed genes, we then log2 transformed the expression data [log2(RSEM+1)], and performed a t -test on gene expression between the normal group and the tumour group for each gene using 254 TCGA colorectal RNA-seq data sets. We selected statistically significant genes that showed a statisically significant twofold change in expression ( P <0.01, after adjustment by Benjamini and Hochberg’s FDR Methods). To generate the heatmap showing expression of genes in the TCGA samples, we log2-transformed the expression data of the 254 TCGA colorectal samples RNA-seq [log2(RSEM+1)]. Then we computed the mean and s.d. of the expression of the each gene ( and s u ). We normalized gene expression by . Hierarchical clustering with Ward’s method was used to normalize TSS/exon gene expression. ChIP-seq analysis Two replicate H3K27Ac ChIP-seq data sets from HCT116 cells (ENCODE accession number wgEncodeEH002873) and two replicate H3K27Ac ChIP-seq data sets from normal sigmoid colon ( www.genboree.org/EdaccData/Current-Release/sampleexperiment/-Sigmoid_Colon/Histone_H3K27ac/ ) were analyzed using the Sole-search ChIP-seq peak calling programme [27] , [28] using the following parameters: Permutation, 5; Fragment, 250; AlphaValue, 0.00010=1.0E−4; FDR, 0.00010=1.0E−4; PeakMergeDistance, 0; HistoneBlurLength, 1,200. Each data set was analyzed separately and also analyzed as a merged data set for HCT116 or sigmoid colon. The merged H3K27Ac peaks from HCT116 or Sigmoid colon were analyzed using the GenomicRanges package of bioconductor to identify promoter versus distal peaks. Enhancer deletion Guide RNAs designed to recognize chr8: 128412821-128412843 and chr8: 128414816-128414838 (hg19) were cloned into a genomic RNA cloning vector (Addgene plasmid 41824) and introduced into HCT116 cells by transfection, along with a plasmid encoding Cas9 and green fluorescent protein. Cells were sorted using a flow cytometer to capture the cells having high green fluorescent protein signals and then colonies were grown from single cells. Complete deletion of all alleles for enhancer 7 was confirmed by PCR using primers flanking the enhancer. RNA analysis was performed in triplicate using HumanHT-12 v4 Expression BeadChip arrays (Illumina), comparing the deleted cells to parental HCT116 cells. Analysis of FunciSNP and correlated SNPs effects To identify SNPs correlated with the 25 CRC tag SNPs and those that overlap with chromatin biofeatures, we use the R package for FunciSNP [21] , which is available in Bioconductor. We used H3K27ac ChIP-seq data from HCT116 cells and sigmoid colon tissue and as biofeatures we used exon, intron, UTR and TSS annotations generated from GENCODE V15. We ran FunciSNP with the following parameters: ±200 kb around each of the 25 tag SNPs and r 2 >0.1. To analyze the potential effects of correlated SNPs on protein coding, we employed SnpEff and Provean using suggested default parameters. For analysis of SNPs on transcription factor motifs, we employ a method developed by Hazelett et al. [58] Batch effects analysis We note that TCGA has strict sample criteria. Each frozen primary tumour specimen has a companion normal tissue specimen which could be blood/blood components (including DNA extracted at the tissue source site), or adjacent normal tissue taken from greater than 2 cm from the tumour. Each tumour and adjacent normal tissue specimen (if available) were embedded in optimal cutting temperature medium and a histologic section was obtained for review. Each haematoxylin and eosin stained case was reviewed by a board-certified pathologist to confirm that the tumour specimen was histologically consistent with colon adenocarcinoma and the adjacent normal specimen contained no tumour cells. The tumour sections were required to contain an average of 60% tumour cell nuclei (TCGA has found that this provides a sufficient proportion so that the tumour signal can be distinguished from other cells), with less than 20% necrosis for inclusion in the study per TCGA protocol requirements. To address potential batch effects, we applied MBatch software, which was developed by the MD Anderson Cancer Center and has been widely used to address batch effects in the TCGA Consortium [2] , [59] , to perform hierarchical clustering and Principal Component Analysis (PCA) to address any potential batch effects in the colorectal TCGA data sets: level 3 mRNA expression (RNA-seq Illumina Hiseq), level 3 DNA methylation (Infinium HM450K microarray), level 4 SNPs copy number variation (CNV) by gene (GW SNP 6). We assessed batch effects for two variables: batch ID and tissue source site. For hierarchical clustering, MBatch uses the average linkage algorithm with 1 minus the Pearson correlation coefficient as the dissimilarity measure. The samples were clustered after labelling with different colours, each of which corresponds to a batch ID or a tissue source site. ( Supplementary Figs 6a.1,6b.1 and 6c.1 ). For PCA, MBatch plotted four principal components ( Supplementary Figs 6a.2,3, 6b.2,3 and 6c.2,3 ). Samples with the same batch ID (or tissue source site) were labelled as same colour and shape and were connected to the batch centroids. The centroids were computed by taking the mean across all samples in the same batch. To assess batch effects on mRNA expression ( Supplementary Fig. 6a ), genes with zero values were removed and normalized gene expression values were log2 transformed before analyzing batch effects. Batch 132 and 154 stood out in one comparison (Comp1 versus Comp2) but not in the other comparisons ( Supplementary Fig. 6a.2 ). The remaining batches or tissue source sites did not stand out in clustering or in any of the PCA plots; thus the data is not supportive of a strong batch effect and all data was used for analysis. When batch effect on CNV ( Supplementary Fig. 6b ) was analyzed, the centroid for the NH tissue source site stood out among other batches. The remaining batches or tissue source sites did not stand out in clustering or in any of the PCA plots. We did not apply correction on the data because (i) there were only two samples and a centroid calculated by only two samples is likely not accurate, (ii) the two samples within the NH batch were not far from other individual samples and (iii) two samples would not dramatically affect our analysis of 233 samples. When assessing batch affects on DNA methylation analysis, no batches or tissue source sites stood out in clustering or in any of the PCA plots. ( Supplementary Fig. 6c ). In summary, none of the samples consistently show batch effects in both clustering and PCA algorithms. Based on the above analysis, we believe that batch effects among the data sets are not dramatically influencing our analysis. eQTL analyses We employed a two-step linear regression model ,which considers somatic germline genotype, CNV and DNA methylation at gene promoters to perform eQTL analysis [60] . We selected 228 patients with both tumour samples and matched normal blood or normal tissue samples from the TCGA CRC data set. For each of these patients, we obtained the germline genotypes from normal blood or normal tissue samples using data from the GW SNP6 array platform. We directly downloaded gene-level somatic copy number, gene isoform expression (from the RNAseqHiseq Illumina platform) and DNA methylation data (from the HM450K platform) for each tumour sample from the TCGA data download website ( http://gdac.broadinstitute.org/runs/analyses__2014_01_15/data/COAD/20140115/ ). To determine DNA methylation of a promoter, we calculated the average DNA methylation at 100 bp upstream of and 700 bp downstream of the TSS for a transcript. We fit the germline genotype of patients, the continuous DNA methylation level of promoters, and the CNV of matched tumour samples into the two-step multivariate linear regression model. Sixty SNPs, including 6 tag SNPs, 18 SNPs within risk enhancers and 45 SNPs within TSS regions, were present on the GW SNP6 array. eQTL analyses were performed using these 60 SNPs and the genes identified by exon or TSS SNPs or by differential expression analysis (see Tables 2 and 5 ). To reduce false positives, we excluded genes showing log2 expression <2 in over 90% of the samples. The Benjamini–Hochberg method was used to correct the original P -value and FDR of 0.1 was used as the threshold of significant association. General data handling and visualization Throughout the analyses we used GenomicRanges to import, export and/or intersect genomic data for plotting and annotation purposes; the R version 3.0.0 (3 April 2013) was used for all statistical analyses, the R function ‘image’ was used for heatmap generation, and package ‘ggplot2’ was used to generate scatterplots. To generate the circle plot, Circos software was used [61] . All genomic location information is based on hg19. How to cite this article: Yao, L. et al. Functional annotation of colon cancer risk SNPs. Nat. Commun. 5:5114 doi: 10.1038/ncomms6114 (2014).